Optically detected cross-relaxation spectroscopy of electron spins in diamond The application of magnetic resonance spectroscopy at progressively smaller length scales may eventually permit ‘chemical imaging’ of spins at the surfaces of materials and biological complexes. In particular, the negatively charged nitrogen-vacancy (NV − ) centre in diamond has been exploited as an optical transducer for nanoscale nuclear magnetic resonance. However, the spectra of detected spins are generally broadened by their interaction with proximate paramagnetic NV − centres through coherent and incoherent mechanisms. Here we demonstrate a detection technique that can resolve the spectra of electron spins coupled to NV − centres, in this case, substitutional nitrogen and neutral nitrogen-vacancy centres in diamond, through optically detected cross-relaxation. The hyperfine spectra of these spins are a unique chemical identifier, suggesting the possibility, in combination with recent results in diamonds harbouring shallow NV − implants, that the spectra of spins external to the diamond can be similarly detected. The negatively charged nitrogen-vacancy (NV − ) centre in diamond has been exploited in optically detected magnetic resonance (ODMR) experiments because of its favourable properties including spin-dependent fluorescence [1] , spin coupling to the magnetic environment [2] and its long polarization lifetime as compared with other similar substrates [3] , even at room temperature. Recent experiments have employed single NV − centres to detect distant nuclear spins in diamond [4] , [5] , [6] , [7] , [8] and external, nanoscale nuclear spin ensembles [9] , [10] , laying the foundations for routine magnetic resonance imaging with nanometre resolution [11] , [12] . Electron spins, in the form of either paramagnetic centres in the diamond lattice or radicals intimately associated with the diamond surface, have also been optically detected through their coupling to the NV − centre [13] , [14] , [15] . The characteristic spectra of the detected spins, however, are often broadened by these same interactions [13] , [14] , [15] . The spectroscopic details are, in general, not sufficiently resolved to provide critical chemical information. One demonstration of optically detected spectroscopy of the electron spin using the NV − centre was performed by sweeping the magnetic field through the cross-relaxation condition between the NV − and the substitutional nitrogen defect (N S ) near ~51.4 mT, where the two electron spin species have commensurate transition frequencies [1] ( Fig. 1a ). However, this method requires frequency matching between allowed transitions in the two spin systems at a specific magnetic field, such that spin flip-flop zero-quantum processes (with Δ m =0, where Δ m is the change of total angular momentum) induced by the dipolar interaction are nearly energy conserved and become allowed; this prevents it from serving as a generic method for optical detection of dark electron or nuclear spins. Frequency matching is only one of many possible conditions that can lead to cross-relaxation [16] ( Fig. 1a ). For instance, cross-relaxation can occur via multiple quantum (for instance, Δ m =±2) spin flip-flop processes that involve the exchange of angular momentum with the lattice, or via multiple spin flips in one system combined with one spin flop in another [16] . Cross-relaxation becomes more obvious at weak magnetic fields, where the difference in the Zeeman energy between spin species is reduced. This is indeed the case for NV − centres in diamond ( Fig. 1b ), as previously suggested by observed dips in the NV − spin-lattice relaxation time ( T 1 ) and by sudden reduction in the optical hole depth (hole bleaching) in the zero-phonon adsorption, in weak magnetic fields (<5 mT) [17] , [18] , [19] , [20] . 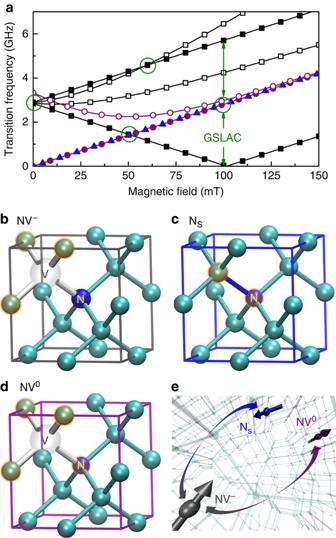Figure 1: Electron spin systems in diamond. (a) Transition frequency of each electron spin system in diamond as a function of the magnetic field. The magnetic field is aligned along one of the NV−axes (solid and open black squares: the NV−centre parallel to and ~109° relative toBz, respectively; solid blue triangles: the NScentre; solid and open purple circles: the NV0centre parallel to and ~109° relative toBz, respectively). The conditions where cross-relaxation occurs are labelled by green circles atBz=0, 51.4, 59.5 and 102.5 mT. (b–d) The structures of the NV−(b), NS(c) and NV0(d) centres. Orange outlines indicate sites at which13C atoms could experience strong hyperfine coupling (>10 MHz) with the corresponding electron spin in the ground states of the NV−and NScentres, or in the4A2excited state of the NV0centre. (e) Illustration of the NV−centre (grey spin symbol) in cross-relaxation with the nearest NScentre (blue spin symbol, ~3 nm away) or NV0centre (purple spin symbol) in diamond. Figure 1: Electron spin systems in diamond. ( a ) Transition frequency of each electron spin system in diamond as a function of the magnetic field. The magnetic field is aligned along one of the NV − axes (solid and open black squares: the NV − centre parallel to and ~109° relative to B z , respectively; solid blue triangles: the N S centre; solid and open purple circles: the NV 0 centre parallel to and ~109° relative to B z , respectively). The conditions where cross-relaxation occurs are labelled by green circles at B z =0, 51.4, 59.5 and 102.5 mT. ( b – d ) The structures of the NV − ( b ), N S ( c ) and NV 0 ( d ) centres. Orange outlines indicate sites at which 13 C atoms could experience strong hyperfine coupling (>10 MHz) with the corresponding electron spin in the ground states of the NV − and N S centres, or in the 4 A 2 excited state of the NV 0 centre. ( e ) Illustration of the NV − centre (grey spin symbol) in cross-relaxation with the nearest N S centre (blue spin symbol, ~3 nm away) or NV 0 centre (purple spin symbol) in diamond. Full size image Here, using a method based on cross-relaxation phenomena in a weak magnetic field, we demonstrate optically detected spectroscopy of electron spins, namely, the N S and neutral nitrogen-vacancy (NV 0 ) centres in diamond ( Fig. 1c,d , respectively), by identifying their respective spectral characteristics in the NV − cross-relaxation ODMR spectrum. This technique is the only demonstrated ODMR method that can provide detailed spectra of the detected electron spins. Such information is essential for the use of the NV − centre for the detection and identification of radicals or relaxation centres, and for the transduction of chemically informative NMR spectra by optical means. Optically detected hyperfine spectra of dark electron spins We demonstrate this technique on an ensemble of NV − centres in a single-crystal diamond, host to several types of paramagnetic defects that may be identified from the ODMR spectra as shown in Fig. 2 (see Methods). The measured spectra have chemically informative fine features that differ vastly from ODMR spectra based on the allowed electron spin transitions of the NV − centre alone [21] , [22] . The majority of the fine features can be assigned to the N S centre [17] , [18] , [20] , [23] (see Supplementary Note 1 ), from which almost all calculated transitions (blue lines on top of each spectrum) are present in the observed spectra. For instance, the three calculated transition frequencies of the N S centre at B z ~0 mT (that is, ambient field), namely, 18.4, 130.2 and 148.6 MHz ( Supplementary Fig. 1c ), are matched with peaks in the ODMR spectrum ( Fig. 2a ). The intensity of the peaks agrees well with the 1:3 population ratio of N S centres oriented either parallel to B z (for example, the peak at 240 MHz in Fig. 2d ) or ~109° relative to B z (the peak at 223 MHz in Fig. 2d ). The observed fine features are also plotted against the calculated hyperfine structure of the N S centre as a function of magnetic field in Fig. 3a . Most of the observed fine features can be assigned to the unique hyperfine structure of the N S centre at various magnetic fields (<5 mT). Although the N S centre is a dark spin whose hyperfine parameters were determined by electron paramagnetic resonance (EPR) [23] , our observations show that the characteristic spectra of the N S centres can also be resolved by ODMR. 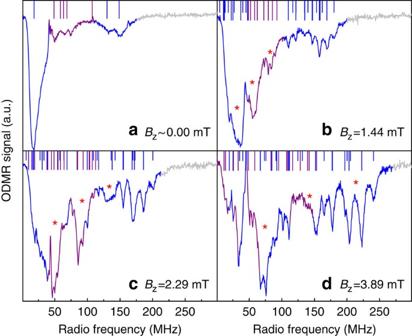Figure 2: ODMR spectra acquired at weak magnetic field. The spectra are acquired at (a)Bz≈0 mT (ambient field), (b)Bz=1.44 mT, (c)Bz=2.29 mT and (d)Bz=3.89 mT. The fine features of the observed spectra are assigned to the NSand NV0centres, which are coloured in blue and purple, respectively. Such assignment is based on the calculated transition frequencies of the NS(blue lines on the top of each spectrum) and NV0(purple lines on the top of each spectrum) centres. All transitions from the NScentre and the relevant transitions of the NV0centre oriented parallel toBzare shown. The short and long blue lines with 1:3 ratio in length correspond to the NScentres oriented parallel toBzand ~109° relative toBz, respectively, with 1:3 ratio in population. The red asterisks (*) represent the difference in transition frequencies between the magnetically inequivalent NV−centres. Figure 2: ODMR spectra acquired at weak magnetic field. The spectra are acquired at ( a ) B z ≈0 mT (ambient field), ( b ) B z =1.44 mT, ( c ) B z =2.29 mT and ( d ) B z =3.89 mT. The fine features of the observed spectra are assigned to the N S and NV 0 centres, which are coloured in blue and purple, respectively. Such assignment is based on the calculated transition frequencies of the N S (blue lines on the top of each spectrum) and NV 0 (purple lines on the top of each spectrum) centres. All transitions from the N S centre and the relevant transitions of the NV 0 centre oriented parallel to B z are shown. The short and long blue lines with 1:3 ratio in length correspond to the N S centres oriented parallel to B z and ~109° relative to B z , respectively, with 1:3 ratio in population. The red asterisks (*) represent the difference in transition frequencies between the magnetically inequivalent NV − centres. 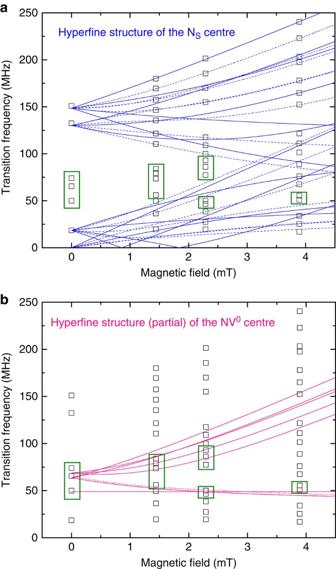Figure 3: Comparison of observed fine features in ODMR spectra with the hyperfine structure of the NSand NV0centres. (a) The majority of fine features (open squares) can be assigned to the hyperfine structure of the NScentre (blue solid lines: the NScentre parallel toBz; blue dashed lines: the NScentre ~109° relative toBz). Several fine features that cannot be assigned to the NScentre are highlighted by green boxes. All possible transitions between the hyperfine structure of the NScentre are shown. (b) The remaining fine features (within green boxes) agree well with the hyperfine structure of the NV0centre (purple solid lines: the NV0centre parallel toBz; purple dashed lines: the NV0centre ~109° relative toBz). For simplicity, only the relevant hyperfine transitions are shown for the NV0centre. Full size image Figure 3: Comparison of observed fine features in ODMR spectra with the hyperfine structure of the N S and NV 0 centres. ( a ) The majority of fine features (open squares) can be assigned to the hyperfine structure of the N S centre (blue solid lines: the N S centre parallel to B z ; blue dashed lines: the N S centre ~109° relative to B z ). Several fine features that cannot be assigned to the N S centre are highlighted by green boxes. All possible transitions between the hyperfine structure of the N S centre are shown. ( b ) The remaining fine features (within green boxes) agree well with the hyperfine structure of the NV 0 centre (purple solid lines: the NV 0 centre parallel to B z ; purple dashed lines: the NV 0 centre ~109° relative to B z ). For simplicity, only the relevant hyperfine transitions are shown for the NV 0 centre. Full size image With the majority of the fine spectral features assigned, there remain some fine features that cannot be matched with the hyperfine structure of the N S centre, as shown in green squares in Fig. 3a . This indicates that we may have observed other defect centres in diamond. The unassigned fine features can be used to identify these additional centres by comparing with the unique hyperfine structures of known defect centres that are commonly found in diamond [24] . We find that the remaining fine features are most consistent with transitions of the NV 0 centre in the spin-3/2 4 A 2 excited state [25] , [26] , [27] (purple lines on top of each spectrum in Fig. 2 , see Supplementary Fig. 1e and Supplementary Note 1 ). For instance, there is an excellent agreement between calculations and the observed transitions at 60, 70, 84 and 92 MHz at 1.44 mT ( Figs 2b and 3b ). These demonstrate that the NV 0 centre is optically detected with part of its characteristic spectrum resolved. As the magnetic field increases above 2 mT, most transitions of the NV 0 centre overlap with those of the N S centre, suggesting that very weak magnetic field is required to separately resolve the two species. The NV 0 centre is a ‘dark state’ of the NV − centre because it requires shorter excitation and detection wavelength than those optimized for NV − centre, and unlike the NV − centre it has not been detected previously using ODMR [27] , [28] , [29] . EPR spectra of the NV 0 centre have been observed only recently for its 4 A 2 exited state under laser illumination [25] . We demonstrate here that the 4 A 2 exited state of the NV 0 centre can also be detected by ODMR via its coupling to the NV − centre. Our observation of the NV 0 centre agrees with the previous characterization of this particular diamond crystal, in which a considerable amount of NV 0 centres have been created along with NV − centres [21] . The ratio of zero-phonon line intensity of NV − and NV 0 was measured to be 3–9 depending on the depth from the diamond surface, after proton irradiation and annealing at 500 °C, and this ratio was shown to remain on the same order of magnitude for subsequent annealing processes [21] . Felton et al. [25] have shown in an EPR experiment that the NV 0 centre is selectively polarized to the sublevel of its spin-3/2 4 A 2 exited state under laser illumination. An optical excitation energy higher than ~2.2 eV (wavelength <563 nm) is required for such polarization [25] , suggesting that the 532 nm laser used in our experiment can also polarize the 4 A 2 exited state of the NV 0 centre. This polarization process of the NV 0 centre starts with the optical excitation from the 2 E ground state to the 2 A 2 excited state [30] , followed by the intersystem crossing from 2 A 2 to 4 A 2 excited state with the details of its mechanism requiring further investigation [30] . The long lifetime of the 4 A 2 excited state allows for detection by EPR measurement [25] . Our observations of the 4 A 2 exited state of the NV 0 centre are consistent with these previous experimental and theoretical studies on the NV 0 centre. The origin of NV 0 -related peaks can potentially be further examined by using orange (wavelength ~593 nm) rather than green light (wavelength ~532 nm) for optical excitation [29] . The former wavelength can maximize ionization (from NV − to NV 0 ) and minimize recombination (from NV 0 to NV − ) such that the majority (~80%) of the NV − centres are in the NV 0 charged state [29] . This can be combined with EPR techniques to improve the precision of the hyperfine structure of the NV 0 centre [25] . However, our instrument is currently not set up to perform either wavelength-dependent excitation or conventional low temperature EPR experiments, and so further investigation is warranted. Cross-relaxation as the optical sensing mechanism The favourable optical and magnetic properties that allow ODMR observation of the NV − centre are known to be absent in the N S and NV 0 centres: the N S centre is a dark spin, while the NV 0 centre is a ‘dark state’ of the nitrogen-vacancy centre and its fluorescence intensity does not depend on the spin state [1] , [27] , [28] , [29] . The radiofrequency (RF)-driven transitions of the N S and NV 0 centres must therefore be sensed by the neighbouring NV − centres to be observed in the ODMR spectra. That is to say, the magnetic resonance of the N S and NV 0 centres are converted into an optical signal by the NV − centre. Such indirectly detected transitions should therefore be a second-order effect compared with the allowed transitions of the NV − centre. This is consistent with the much smaller (~1/60) optical contrast of the observed hyperfine features compared with that of the allowed NV − transitions. On the other hand, the fine features of the N S and NV 0 centres are observed at the frequencies of their own hyperfine structure, far below the allowed transition frequencies of the NV − centre. This suggests that the N S and NV 0 centres are instead perturbing seemingly ‘forbidden’ transitions, for instance, the transition between the |+1〉 and |−1〉 sublevels of the NV − centre. Such perturbation is possible because there is indeed an energy match between the hyperfine levels of the N S (or NV 0 ) and the |+1〉↔|−1〉 sublevels of the NV − centre [17] . Although the |+1〉↔|−1〉 transition cannot be directly induced by application of microwaves (MWs) due to the selection rule (Δ m S =±1), cross-relaxation between the NV − and N S centres via the |+1〉 and |−1〉 sublevels at weak magnetic field is an established process that has been thoroughly studied, both experimentally and theoretically [17] , [18] , [31] , [32] , [33] , [34] . Cross-relaxation can occur among almost any two spin systems as long as there is an energy matching condition, such as between two subensembles of NV − centres at zero field, between the NV − and N S centres at weak magnetic field, and between magnetically inequivalent or equivalent NV − centres at certain values of the strength and angle of the applied magnetic field [17] , [18] , [31] , [32] , [33] , [34] . Cross-relaxation between two spin systems occurs when energy exchange between two systems provides additional spin-lattice relaxation pathways for both systems. The signature of cross-relaxation can be verified by perturbing the relaxation process of one spin system while monitoring the relaxation response (that is, the change in T 1 ) of the other system. The fact that we observe the characteristic hyperfine spectra of N S and NV 0 centres within the ODMR continuous-wave (CW) spectra of NV − centres is thus a signature of cross-relaxation. First, the applied RF drives the hyperfine transitions of N S and NV 0 centres only (as it is off-resonance for NV − allowed transitions). Second, the ODMR signal comes solely from the NV − centres because both N S and NV 0 are ‘dark’ under the experimental conditions [1] , [27] , [29] , and the optical signal (steady-state fluorescence intensity) is directly related to the T 1 of the NV − centres [1] . We therefore altered the relaxation response of NV − centres by perturbing the relaxation process of N S or NV 0 centres. More specifically, the energy matching condition required by cross-relaxation is satisfied between the |+1〉 and |−1〉 sublevels of the NV − centres and the hyperfine levels of the N S or NV 0 centres. The spin flip-flop processes between NV − and N S (or NV 0 ) centres can thus be induced by the dipolar interaction between them, which couples the two spin systems via efficient energy exchange and leads to cross-relaxation. Here we must point out that cross-relaxation via the |+1〉 and |−1〉 sublevels of the NV − centres will result in a decrease in the steady-state fluorescence intensity ( Supplementary Note 2 ). Since the |0〉 sublevel of the NV − centre is the ‘brighter’ state, a relative population change between |+1〉 and |−1〉 sublevels will not directly lead to a change in fluorescence intensity. However, while the ODMR CW spectra are acquired, the processes of optical pumping towards the |0〉 sublevel and relaxation back to the |±1〉 sublevels reach equilibrium. When cross-relaxation occurs via the |+1〉 and |−1〉 sublevels, a different equilibrium condition will be established, resulting in lower population on the |0〉 sublevel and thus a decrease in fluorescence intensity ( Supplementary Equations 4–7 in Supplementary Note 2 ). This occurs because the continuous optical pumping process couples together the populations of all three sublevels of the NV − centre, and enhanced relaxation between the |+1〉 and |−1〉 sublevels will affect the population on the |0〉 sublevel as well ( Supplementary Note 2 ). Such a phenomenon has been observed in experiment, and the cross-relaxation mechanism has been suggested as well [17] . This is different from the pulsed ODMR experiment, in which the polarization is optically initialized first, and then MW irradiation is used to manipulate the populations of different sublevels; the steady-state condition in the CW experiment ceases to exist when the optical pumping cycle is turned off. Furthermore, when the spin transition between two hyperfine levels of the N S or NV 0 spin system is driven by resonant RF, the spin-lattice relaxation of the NV − spin will be further enhanced (that is, T 1 is shortened) by cross-relaxation. As a result, the fluorescence intensity of the NV − centre decreases [1] , [18] , [29] , leading to the observed ODMR peaks as shown in Fig. 2 , serving as the basis for cross-relaxation spectroscopy. Here, the resonant RF only affects the N S or NV 0 spins, while the laser irradiation and optical detection occur through the NV − centres ( Fig. 4 ). The cross-relaxation provides an effective energy exchange between the spin systems and serves as a generic mechanism to convert the magnetic resonance of N S and NV 0 spins into changes in optical signal of the NV − centre. 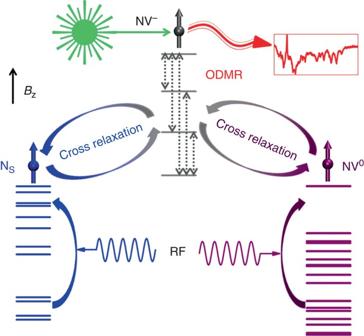Figure 4: Schematic illustration of optically detected cross-relaxation spectroscopy. Cross-relaxation occurs between the NV−and NScentres, between the NV−and NV0centres and between magnetically inequivalent NV−centres. When one of the NSor NV0transitions is saturated by RF radiation, the fluorescence intensity of the NV−centres decreases, resulting in the observed ODMR spectra. Figure 4: Schematic illustration of optically detected cross-relaxation spectroscopy. Cross-relaxation occurs between the NV − and N S centres, between the NV − and NV 0 centres and between magnetically inequivalent NV − centres. When one of the N S or NV 0 transitions is saturated by RF radiation, the fluorescence intensity of the NV − centres decreases, resulting in the observed ODMR spectra. Full size image Cross-relaxation among NV − centres In addition to the fine features in the ODMR spectra, relatively broad peaks with full-width at half-maximum (FWHM) of ~20 MHz are also observed. The central frequency of each broad peak agrees well with the calculated energy difference between magnetically inequivalent NV − centres (different orientations either parallel to B z or ~109° relative to B z ) or between neighbouring magnetically equivalent NV − centres (both parallel to B z ). The calculated energy difference is labelled by asterisks in Fig. 2 ( Supplementary Fig. 1a and Supplementary Note 1 ). For instance, in Fig. 2b , the middle broad peak at ~54 MHz matches the energy difference between the |+1〉 sublevel of NV − parallel to B z and the |−1〉 sublevel of NV − ~109° relative to B z (or vice versa), suggesting that cross-relaxation occurs between magnetically inequivalent NV − centres. This can be further verified, as will be shown later, owing to the different resonance frequencies for the magnetically inequivalent NV − centres. The FWHM here (~20 MHz) is approximately twice the FWHM of the peaks associated with allowed transitions in ODMR spectra (~10 MHz, see Fig. 5 ), providing additional evidence that the applied RF matches the energy difference between two NV − centres. Here, the RF enhances cross-relaxation by providing the energy difference between two NV − centres, which otherwise need to exchange energy via phonons [35] . This effect is different from the cross-relaxation between NV − and N S (or NV 0 ) centres, in which RF provides the energy cost for N S (or NV 0 ) transitions, and the energy cost for NV − -N S or NV − -NV 0 spin flip-flop processes is taken from the lattice. In both cases, the RF is applied to provide the energy required for efficient cross-relaxation process. 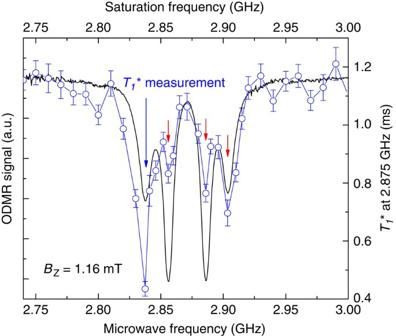Figure 5: Cross-saturation among magnetically inequivalent NV−centres. Cross-saturation between NV−centres with different orientations, either parallel toBzor ~109° relative toBzatBz=1.16 mT. The thick black line shows the ODMR spectrum (left and bottom axes) acquired near ~2.87 GHz, where the allowed transitions of NV−centres at different orientations can be resolved. The effective longitudinal relaxation time(scatter data with error bars representing the s.d., right and top axes) is measured at 2.8375 GHz (blue arrow), the frequency of the |0〉↔|−1〉 transition of the NV−centres oriented parallel toBz, while saturating another MW frequency. The change inis well correlated with the ODMR spectrum;is significantly reduced (red arrows) when the saturating frequency is resonant with the transitions of the NV−centres oriented ~109° relative toBz, or with the |0〉↔|+1〉 transition of the NV−centres oriented parallel toBz. Figure 5: Cross-saturation among magnetically inequivalent NV − centres. Cross-saturation between NV − centres with different orientations, either parallel to B z or ~109° relative to B z at B z =1.16 mT. The thick black line shows the ODMR spectrum (left and bottom axes) acquired near ~2.87 GHz, where the allowed transitions of NV − centres at different orientations can be resolved. The effective longitudinal relaxation time (scatter data with error bars representing the s.d., right and top axes) is measured at 2.8375 GHz (blue arrow), the frequency of the |0〉↔|−1〉 transition of the NV − centres oriented parallel to B z , while saturating another MW frequency. The change in is well correlated with the ODMR spectrum; is significantly reduced (red arrows) when the saturating frequency is resonant with the transitions of the NV − centres oriented ~109° relative to B z , or with the |0〉↔|+1〉 transition of the NV − centres oriented parallel to B z . Full size image An additional broad peak at ~28 (or ~81) MHz in Fig. 2b matches the energy difference between the |+1〉 sublevel of one NV − and the |−1〉 level of another NV − in close proximity, both of which are ~109° relative to B z (or both parallel to B z ). It is likely that cross-relaxation between magnetically equivalent NV − centres is the dominant mechanism for these peaks. This, however, cannot be further verified because the magnetically equivalent NV − centres have identical resonance frequencies, and neighbouring centres thus cannot be separately addressed. There could also be contributions from the small mixing between |0〉 and |±1〉 sublevels that makes the |−1〉↔|+1〉 transition weakly allowed and causes a small optical contrast. Nevertheless, the three broad features have near equal intervals because the energy levels of neighbouring NV − centres, either magnetically inequivalent or equivalent, are nearly evenly spaced ( Supplementary Fig. 1a ). The hyperfine interaction with 13 C is not considered here because only about 3.3% of the NV − centres experience strong hyperfine interaction (~130 MHz) with a first-shell 13 C. For the majority of the NV − centres in the ensemble, hyperfine interaction with 13 C causes line broadening with little effect on the central frequency. Cross-relaxation between magnetically inequivalent NV − centres can be directly observed by measuring the spin-lattice relaxation time of the NV − centre parallel to B z , while saturating either the transition of the NV − centre ~109° relative to B z , or the other allowed transitions of the NV − centre parallel to B z (see Methods). Figure 5 shows the apparent spin-lattice relaxation time ( ), measured at the |0〉↔|−1〉 transition frequency of the NV − centres oriented parallel to B z , as a function of the saturation MW frequency. The apparent relaxation time becomes much shorter when the saturation frequency is on resonance with either the allowed transitions of the NV − centres ~109° relative to B z , or with the |0〉↔|+1〉 transition of the NV − centres parallel to B z . These observations provide direct evidence that there is cross-relaxation among the NV − centres. Since cross-relaxation is reciprocal, the apparent relaxation time measured at the frequency of any one of the four peaks in CW spectra will become shorter when the saturation frequency is tuned to the frequency of another peak. Note that saturation of dark electron spin transitions does not cause an observable change in the of the NV − centres because of the relatively low polarization of the N S and NV 0 centres. Cross-relaxation at the ground state-level anti-crossing Additional evidence to support the claim that cross-relaxation is the conversion mechanism from magnetic resonance to optical signal is supplied by an investigation of spectra at other known conditions at which cross-relaxation occurs. It is known that cross-relaxation occurs near the ground state-level anti-crossing (GSLAC) at ~102.5 mT (ref. 17 ), where the |0〉 and |−1〉 sublevels of the NV − centre approach degeneracy and the |0〉↔|+1〉 transition frequency of the NV − centre is almost twice the transition frequencies of the N S and NV 0 centres ( Fig. 1a ). This cross-relaxation can occur through a NV − flip paired with the flops of two electron spins, with the balance of the angular momentum transferred to the rigid lattice [16] . The applied resonant MW radiation induces transitions between energy levels of the N S and NV 0 centres, which indirectly affects the NV − centre via cross-relaxation. The cross-relaxation process itself is governed by the mutual interaction between spins, and thus is not directly affected by the applied MW. The characteristic peaks of the N S and NV 0 centres are clearly resolved and identified in the ODMR spectrum within the 2.7–3.0 GHz range ( Fig. 6 ). Four possible orientations of the N S centres lead to two triplets (blue bars on the bottom of the spectrum in Fig. 6 ) with overlapping central peaks when the external field is aligned with one of the N S (or NV − ) symmetry axes [1] , [15] , [36] . The remaining peaks agree well with the calculated transition frequencies of NV 0 centres oriented parallel to B z ; discrepancies and unassigned peaks may be due to the accuracy of the available quadrupolar interaction parameters [27] , and the zero-field splitting and hyperfine interaction parameters that were determined for the 15 NV 0 system at the spin-3/2 4 A 2 excited state [25] . Although the sublevels of the NV 0 4 A 2 excited state are selectively polarized, the direct transition between them has not been observed by EPR, probably because it is obscured by other paramagnetic centres in diamond [25] . Near GSLAC, the nearly complete electron spin polarization of the NV − centres can be transferred to the neighbouring electron spins via their mutual interactions, resulting in greater polarization [36] and thus greater signals from the N S and NV 0 electron spins, similar to observations at the cross-relaxation condition near ~51.4 mT [1] . Thus far, the hyperfine features of the N S and NV 0 centres in ODMR spectra are observed at two separate cross-relaxation conditions (that is, weak magnetic field and GSLAC). This confirms that the cross-relaxation serves as the sensing mechanism by converting magnetic resonance of the N S and NV 0 centres to an optical signal produced by the NV − centre. 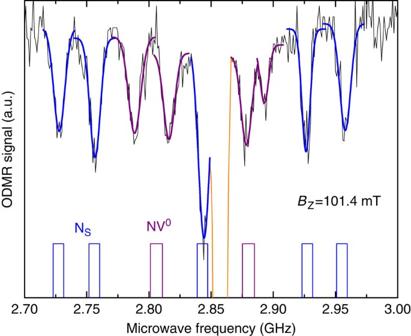Figure 6: ODMR spectrum near GSLAC. The ODMR spectrum is acquired atBz=101.4 mT. The most intense peak, centred at ~2.857 GHz and coloured orange, is an artefact whose second harmonic matches the frequency of the |0〉↔|+1〉 ground state transition of the NV−centre parallel toBz. Each resolved side peak is fitted into a Gaussian function and assigned to either the NScentre (blue curves) or the NV0centre (purple curve). The assignment is based on the calculated transition frequencies of each centre and its respective Hamiltonian, as shown by the vertical bars at the bottom. All allowed transitions of the NScentre in the ground state are clearly resolved at the predicted transition frequencies (blue bars). The rest of the observed side peaks are consistent with thetransitions of the NV0centre in the4A2exited state with discrepancies from the predicted transition frequencies (purple bars) probably due to the accuracy of the available spin Hamiltonian parameters. Figure 6: ODMR spectrum near GSLAC. The ODMR spectrum is acquired at B z =101.4 mT. The most intense peak, centred at ~2.857 GHz and coloured orange, is an artefact whose second harmonic matches the frequency of the |0〉↔|+1〉 ground state transition of the NV − centre parallel to B z . Each resolved side peak is fitted into a Gaussian function and assigned to either the N S centre (blue curves) or the NV 0 centre (purple curve). The assignment is based on the calculated transition frequencies of each centre and its respective Hamiltonian, as shown by the vertical bars at the bottom. All allowed transitions of the N S centre in the ground state are clearly resolved at the predicted transition frequencies (blue bars). The rest of the observed side peaks are consistent with the transitions of the NV 0 centre in the 4 A 2 exited state with discrepancies from the predicted transition frequencies (purple bars) probably due to the accuracy of the available spin Hamiltonian parameters. Full size image Our cross-relaxation spectroscopy technique generically detects the spectra of electron spins using the NV − centre ( Fig. 4 ). The steady-state fluorescence intensity of the NV − centre is directly observed without requiring the creation or manipulation of NV − spin coherences as in other methods. This effectively moves the detection of electron spins from the indirect to the direct frequency dimension, thereby improving both frequency resolution and detection sensitivity. Detection is no longer limited by the coherence time of the NV − centre, and as a result much longer detection times can be used to improve the signal-to-noise ratio. The fine frequency resolution and high sensitivity of this technique may also allow the identification of additional unknown paramagnetic centres that have been obscured by the N S centre in EPR [25] measurements, in a similar manner to our detection of the NV 0 centre. These results provide an optically detected analogue of nuclear magnetic cross-relaxation spectroscopy in solid and dilute spin systems [37] , [38] . It may also be possible to use cross-relaxation spectroscopy for detection of electron spins external to the diamond sample. The potential detection distance through cross-relaxation should be at least ~8 nm, as estimated by the average separation of neighbouring NV − centres in our diamond sample, between which cross-relaxation is clearly detected in our measurements [39] ( Supplementary Note 3 ). Such a detection distance would allow for observation and identification of dark electron spins deposited on the diamond surface [14] , if using shallow-implanted NV − centres in ultrapure diamond [3] , [40] . For that purpose, ultrapure diamond with much lower N S centre concentrations must be used to remove the background hyperfine features from the N S impurities in diamond. The optically detected spectra of radicals via NV − centres can be used to determine chemical identity by comparing with a database of characteristic hyperfine structures of known radicals, a process similar to existing EPR methods for determining hyperfine constants of a radical. In Supplementary Fig. 3 , we consider as an example the free radical diphenyl picryl hydrazyl ( Supplementary Note 4 ), which has hyperfine structures vastly different from the detected centres in diamond [41] , [42] . Furthermore, radicals on the diamond surface could be used as a detection intermediate for external nuclear spins located at even further distances [43] ; an ensemble of radicals of a single type could significantly increase the detected magnetic flux [44] , while spatially engineered arrays of radicals of different species could provide spatial resolution for detection of distant nuclear spins or simply act as a gradiometer [15] , [45] . Materials and experiments The diamond sample used in our experiments was fabricated commercially by Element-6 using high-pressure high-temperature synthesis. It was then irradiated, annealed and characterized as previously reported [21] , [45] , where it was labelled as sample S9. The diamond sample has been shown to contain NV − centres (up to ~2 p.p.m. in the most dense location), N S centres (~50 p.p.m.) and NV 0 centres (NV − : NV 0 =3–9, depending on the depth from the diamond surface) [21] . The average distance between nearest NV − centres is ~8 nm and that between an NV − centre and the nearest N S centre is ~3 nm, as estimated by the Poisson distribution for the typical distance between neighbouring particles [46] . The ODMR apparatus was described in detail elsewhere [22] and we only briefly describe it here. A continuous beam from a 532-nm laser with optical power of 2 mW is focused on the diamond by an objective lens with a numerical aperture of 0.7 to achieve optical power density of ~5 mW μm −2 . The fluorescence signal from the NV − is collected by an avalanche photo detector after passing a dichroic mirror and a long-pass filter [45] . The external magnetic field is applied using a permanent magnet aligned to one of the NV − symmetry axes, with the field strength adjusted by the magnet’s distance to the diamond and determined using the NV − centres as a magnetometer [21] , [22] . The RF radiation is swept from 1 to 300 MHz using a single copper wire loop to produce an oscillating magnetic field of ~0.1 mT in amplitude. The ODMR CW spectra record the steady-state fluorescence intensity under conditions of continuous RF excitation, compared with that with RF turned off for reference. The spectra are averaged over 2,000 scans. In the double resonance experiments, pulsed MW excitation is delivered using the same copper wire loop, while continuous MW radiation is applied with an additional copper wire to saturate additional transitions. A standard inversion recovery sequence is used to measure the change in at the |0〉↔|−1〉 transition frequency of the NV − centres oriented parallel to B z , while saturating transitions of the NV − centres oriented ~109° relative to B z at a different MW frequency. How to cite this article: Wang, H.-J. et al. Optically detected cross-relaxation spectroscopy of electron spins in diamond. Nat. Commun. 5:4135 doi: 10.1038/ncomms5135 (2014).